A micro-sterile inflammation array as an adjuvant for influenza vaccines There is an urgent need of adjuvants for cutaneous vaccination. Here, we report that micro-sterile inflammation induced at inoculation sites can augment immune responses to influenza vaccines in animal models. The inoculation site is briefly illuminated with a handheld, non-ablative fractional laser before the vaccine is intradermally administered, which creates an array of self-healing microthermal zones (MTZs) in the skin. The dying cells in the MTZs send ‘danger’ signals that attract a large number of antigen-presenting cells, in particular, plasmacytoid dendritic cells (pDCs) around each MTZ forming a micro-sterile inflammation array. A pivotal role for pDCs in the adjuvanticity is ascertained by significant abrogation of the immunity after systemic depletion of pDCs, local application of a TNF-α inhibitor or null mutation of IFN regulatory factor7 (IRF7). In contrast to conventional adjuvants that cause persistent inflammation and skin lesions, micro-sterile inflammation enhances efficacy of influenza vaccines, yet with diminished adverse effects. We have made tremendous progress in the past decade in understanding sterile inflammation, which is induced by danger signals released from dying cells as a natural response to invaders or injuries to protect our body [1] . The danger signals, known as damage-associated molecular patterns, include uric acid, dsDNA, RNA and others, and they can attract and activate antigen-presenting cells (APCs). The sterile inflammation is one of the primary mechanisms behind aluminium salt, also called alum, and MF59 adjuvants, two licensed vaccine adjuvants, and forms the basis for today’s adjuvant development [2] , [3] , [4] , [5] , [6] . The ability of sterile inflammation to augment immune responses against vaccines raises an intriguing possibility that skin injury can serve as an ‘adjuvant’ for cutaneous vaccination, provided that the injury is well under control. Non-ablative fractional laser (NAFL) can controllably injure the dermis at the site of vaccine inoculation. The laser treatment generates an array of self-renewable microthermal zones (MTZs) in a desirable number, size and depth without damaging skin’s outer protective layer, so that skin barrier function can be well preserved [7] . Each MTZ is so small that it can heal within days by fast-growing epithelial cells surrounding each MTZ, resulting in younger-looking skin [7] , [8] , [9] , [10] . NAFL technology is a mature industry for dermatologic treatment applications [7] . The micro-skin injury sharply contrasts with the injury induced by intradermal (ID) injection of adjuvants that often evokes severe and persistent inflammation and overt skin lesions, making them not acceptable for routine vaccination [11] . However, whether this fast healing micro-injury in the skin is sufficient to strengthen immune responses has not been yet explored. Skin is prone to adjuvant-induced inflammation, which causes severe local reactogenicity including erythema, swelling and ulceration that can persist for weeks [11] . Because of these unwanted adverse events, most current adjuvants such as alum, oil-in-water emulsion adjuvants and several agonists of Toll-like receptor (TLR) are not suitable for skin vaccination [11] . If we are to take advantages of cutaneous vaccination as a more efficient route over conventional intramuscular (IM) immunization, effective adjuvants that do not cause overt skin inflammation are an urgent need [12] , [13] , [14] , [15] . We present here that NAFL induces sterile inflammation at a micro-scale that causes no overt skin lesions while greatly augmenting immune responses to influenza vaccines ID administered. The danger signals released by dying cells in laser-generated MTZs preferably attract plasmacytoid dendritic cells (pDCs) that are subsequently activated by topically applied imiquimod (IMIQ) cream, an agonist for TLR-7 (ref. 16 ), leading to synergistic augmentation of the immune response against influenza vaccine in adult and old mice as well as in pigs. NAFL/IMIQ adjuvant augments vaccine-induced immune responses An over-the-counter, handheld, cosmetic NAFL generated a 6 × 9 array of 54 MTZs, in a 7 mm × 10 mm rectangular area of the skin as illustrated in Supplementary Fig. 1a,b . Each MTZ was a thermal injury about the size and shape of a hair, approximately 200 μm in diameter and 300 μm in depth. The MTZs heal quickly, giving rise to new and younger skin [17] . The sterile inflammation induced by laser-damage cells was restricted around each MTZ, leaving a majority of tissues unaffected, warranting a quick resolution of the inflammation. To test whether this transient, micro-scale inflammation was sufficient to augment immunity stimulated by various vaccines, a clinical H1N1 influenza vaccine (A/California/7/2009) was ID inoculated into the site of laser illumination. As shown in Fig. 1a , hemagglutinin inhibition (HAI) antibody titres were significantly higher in the presence as compared with the absence of laser treatment ( P <0.05, analysis of variance (ANOVA)/Bonferroni). There was a slightly greater immune response evoked with ID than IM immunization, similar to previous investigations ( Fig. 1a ) (refs 12 , 13 , 18 ). Comparable results were also attained with the protein model antigen ovalbumin, hepatitis B surface antigen vaccine or recombinant influenza hemagglutination (HA) protein, raising specific antibody titres by six- ( P <0.001, t -test), ten- ( P <0.05, t -test) and threefold ( P <0.01, t -test), respectively ( Supplementary Fig. 1c,d,e ). The adjuvant effect of NAFL was primarily ascribed to laser-mediated cell damage. Hence, when influenza vaccine was mixed with a small number of heat (65 or 95 °C)-damaged skin cells and ID administered, the heat-damaged cells enhanced immune responses against the co-injected influenza vaccine at a level comparable to that of laser treatment ( P <0.01 for 65 °C and P <0.05 for 95 °C, ANOVA/Bonferroni, Supplementary Fig. 2 ). Moreover, the laser illumination conferred similar adjuvant effects as that of topic IMIQ cream (Aldara, 3 M Pharmaceuticals), which is a Food and Drug Administration (FDA)-approved topical drug for treatment of some skin diseases ( Fig. 1a ) (ref. 19 ). Strikingly, when laser-treated skin was inoculated with the influenza vaccine, followed by topical application of IMIQ cream, the combination synergistically enhanced HAI titres by sevenfold or fourfold over IM or ID vaccination, respectively ( Fig. 1a , P <0.001, ANOVA/Bonferroni). This robust response was greater than that induced by IM immunization of a 10 × higher amount of the vaccine, suggesting at least 10 × dose-sparing over the current IM influenza vaccination ( Fig. 1a ). Similar trends were attained in total serum IgG and IgA levels ( Fig. 1b,c ). The adjuvant effect was also confirmed in outbred Swiss Webster mice in which IgG and HAI titres were greatly higher with laser pre-illumination than without the illumination ( Supplementary Fig. 3 ). 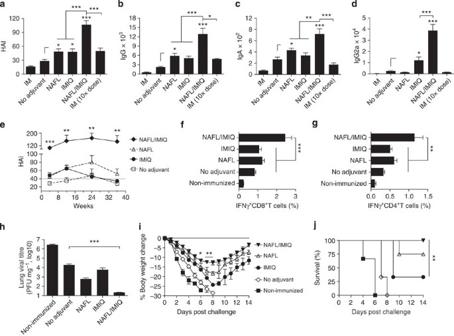Figure 1: NAFL/IMIQ strengthens immunogenicity of ID influenza vaccine. BALB/c mice were ID immunized with 0.06 μg (HA content) H1N1 influenza vaccine alone (no adjuvant) or in the presence of NAFL, IMIQ or NAFL/IMIQ adjuvant or IM immunized with a same dose (IM) or a 10 × higher dose (0.6 μg) of the vaccine. Humoral immune responses were measured 4 weeks later including HAI titre (a), IgG (b), IgA (c) or IgG2a (d). HAI titres were further monitored at 4, 12, 24 and 36 weeks post immunization (e). A horizontal grey line indicates a standard protective titre of HAI.n=8, except for NAFL and NAFL/IMIQ groups (n=10). (f,g) Cell-mediated immune responses. Peripheral blood mononuclear cells were isolated 1 week after immunization, stimulated with the vaccine and anti-CD28 antibody and analysed for the percentages of IFNγ-secreting CD8+(f) and CD4+(g) T cells by flow cytometry.n=6, except for NAFL and NAFL/IMIQ groups (n=8). (h–j) Challenge studies. The immunized mice and non-immunized controls were intranasally challenged with 10 × LD50of A/California/7/2009 H1N1 virus 5 weeks post immunization. The infected mice were euthanized 4 days post infection to determine lung viral titres by TCID50assays using MDCK cells (h).n=6. Body weight (i) and survival (j) were monitored daily for 14 days. Percentages of body weight dropped relative to a pre-infection level and percentages of survival were compared between NAFL/IMIQ and NAFL or IMIQ groups byt-test or Logrank test respectively.n=6, except for NAFL and NAFL/IMIQ groups (n=8). Data are presented as mean±s.e.m. Statistical significance was analysed by ANOVA/Bonferroni unless noted otherwise. *P<0.05; **P<0.01 or ***P<0.001, respectively. All experiments were repeated twice with similar results. Figure 1: NAFL/IMIQ strengthens immunogenicity of ID influenza vaccine. BALB/c mice were ID immunized with 0.06 μg (HA content) H1N1 influenza vaccine alone (no adjuvant) or in the presence of NAFL, IMIQ or NAFL/IMIQ adjuvant or IM immunized with a same dose (IM) or a 10 × higher dose (0.6 μg) of the vaccine. Humoral immune responses were measured 4 weeks later including HAI titre ( a ), IgG ( b ), IgA ( c ) or IgG2a ( d ). HAI titres were further monitored at 4, 12, 24 and 36 weeks post immunization ( e ). A horizontal grey line indicates a standard protective titre of HAI. n =8, except for NAFL and NAFL/IMIQ groups ( n =10). ( f , g ) Cell-mediated immune responses. Peripheral blood mononuclear cells were isolated 1 week after immunization, stimulated with the vaccine and anti-CD28 antibody and analysed for the percentages of IFNγ-secreting CD8 + ( f ) and CD4 + ( g ) T cells by flow cytometry. n =6, except for NAFL and NAFL/IMIQ groups ( n =8). ( h – j ) Challenge studies. The immunized mice and non-immunized controls were intranasally challenged with 10 × LD 50 of A/California/7/2009 H1N1 virus 5 weeks post immunization. The infected mice were euthanized 4 days post infection to determine lung viral titres by TCID 50 assays using MDCK cells ( h ). n =6. Body weight ( i ) and survival ( j ) were monitored daily for 14 days. Percentages of body weight dropped relative to a pre-infection level and percentages of survival were compared between NAFL/IMIQ and NAFL or IMIQ groups by t -test or Logrank test respectively. n =6, except for NAFL and NAFL/IMIQ groups ( n =8). Data are presented as mean±s.e.m. Statistical significance was analysed by ANOVA/Bonferroni unless noted otherwise. * P <0.05; ** P <0.01 or *** P <0.001, respectively. All experiments were repeated twice with similar results. Full size image In humans, a majority of people are primed with influenza viral antigens either via vaccination or natural infections. To test if the NAFL or NAFL/IMIQ adjuvant could boost the immune response efficiently in antigen-primed subjects, mice were primed with H1N1 influenza vaccine with or without NAFL or NAFL/IMIQ, followed by an immunization booster 2 weeks later. As expected, the adjuvant boosted the immune response in primed subjects as effectively as in naïve ones, regardless of whether the primary vaccination was given influenza vaccine alone or the vaccine in combination with NAFL or NAFL/IMIQ adjuvant ( Supplementary Fig. 4 ). Measurement of serum IgG1 and IgG2a antibody titres revealed Thl-skewed immune responses in the presence of NAFL/IMIQ adjuvant. The adjuvant elevated IgG2a production by 15-fold, and only a fivefold increase was seen with IMIQ alone ( Fig. 1d , P <0.001, ANOVA/Bonferroni). In contrast, NAFL alone stimulated mainly IgG1 production with barely detectable IgG2a, indicative of Th2 immune responses. Apparently, topical application of IMIQ cream on the NAFL-treated site is not simply a combination of Th2 and Th1 responses, rather converting it into a stronger Th1 immune response that is required for more effective protection against viral infection ( Supplementary Fig. 5a,b ). The superior humoral immune response at a high HAI titre of more than 1:100 was sustained for at least 9 months without any sign of decline ( Fig. 1e ), a period of time longer than an influenza season which typically lasts for 6 months in the most part of the world. NAFL alone was also able to retain a HAI titre above the standard protective level (1:40) for more than 9 months ( Fig. 1e ). In comparison, topical IMIQ was not as strong as NAFL in sustaining HAI production, and the HAI titre started to decline after 3 months of immunization and reached similar levels as non-adjuvanted influenza vaccine three more months later ( Fig. 1e ). Alongside, the IgG level in NAFL/IMIQ group was also substantially higher than that of other groups throughout the entire experimental period ( Supplementary Fig. 5c ). Not only humoral, but cellular immune responses were also greatly improved by NAFL/IMIQ adjuvant. The percentages of CD8 + and CD4 + T cells secreting IFN-γ in the periphery were vigorously increased only in the NAFL/IMIQ group among all groups tested after influenza viral stimulation ( Fig. 1f,g , P <0.001 or 0.01 ANOVA/Dunnett’s). Enhanced protection against viral infection The immunized mice were challenged with a mouse-adapted A/California/7/2009 H1N1 virus. The NAFL/IMIQ adjuvant greatly reduced lung viral titre to 2.2 × 10 1 plaque-forming unit (PFU) per 1 mg tissue ( P <0.001, ANOVA/Bonferroni), which was 1,000 times lower than that attained in mice receiving the vaccine alone ( Fig. 1h ). Moreover, the body weight dropped by more than 17% in 8 days post infection in all groups except for the NAFL/IMIQ group ( Fig. 1i ). The latter showed a decline in their body weight at the slowest pace, yet recovered at the fastest pace ( Fig. 1i ). All mice died within 8 days in non-immunized controls or mice immunized similarly without any adjuvant ( Fig. 1j ). Four out of six mice died in IMIQ group and two out of eight died in the NAFL group, whereas all mice survived in the NAFL/IMIQ group ( Fig. 1j ). Similar results were obtained in Swiss Webster mice showing substantial reduction of influenza viral replication in the lung of animals immunized with H1N1 influenza vaccine in the presence of the NAFL/IMIQ adjuvant as compared to the vaccine alone ( Supplementary Fig. 3c , P <0.001, ANOVA/Bonferroni). Comparisons between NAFL/IMIQ and a squalene-based adjuvant NAFL/IMIQ adjuvant was further compared with AddaVax (Invivogen), which has a similar formulation and physical/chemical feature as MF59 (ref. 4 ). IM inoculation of influenza vaccine emulsified with an equal amount of AddaVax provoked immune responses slightly inferior to those of the NAFL/IMIQ adjuvant, as measured by IgG and HAI titres ( Fig. 2a,b ), suggesting that the laser-based adjuvant is equal to or somewhat better than this specific squalene-based adjuvant in augmentation of influenza vaccines. However, NAFL/IMIQ caused no overt skin lesions at the inoculation site, although mild inflammation was noticed in 1 day and disappeared within 3 days with histological examination ( Fig. 2c right panel). Similar to previous investigation [17] , small-diameter, thermally coagulated columns were generated in dermis by the laser, with intact stratum corneum and epidermis in place ( Fig. 2c right panel). In contrast, IM administration of AddaVax mixed with influenza vaccine caused inflammation that persisted for more than 1 week ( Fig. 2c left panel). Moreover, NAFL/IMIQ induced a much lower level of proinflammatory cytokine responses systemically as manifested by a relatively lower level of circulating interleukin-6 (IL-6), an important mediator of fever ( Fig. 2d ). IL-6 concentration peaked after 8 h of immunization and reached as high as 134 pg ml −1 in mice receiving the squalene-adjuvanted influenza vaccine, which was four times higher than the 32 pg ml −1 IL-6 seen in mice immunized by the same amount of vaccines with the NAFL/IMIQ adjuvant ( Fig. 2d , P <0.01 t -test). Besides, the squalene-adjuvanted vaccine elevated the body temperature by 1 °C that lasted for 9 h, when compared with mice receiving the vaccine alone ( Fig. 2e ). In sharp contrast, no fever was measurable over the influenza vaccine alone in the NAFL/IMIQ group ( Fig. 2e ). The safety profile requires further confirmation with licensed MF59 in place of commercial AddaVax in future study. 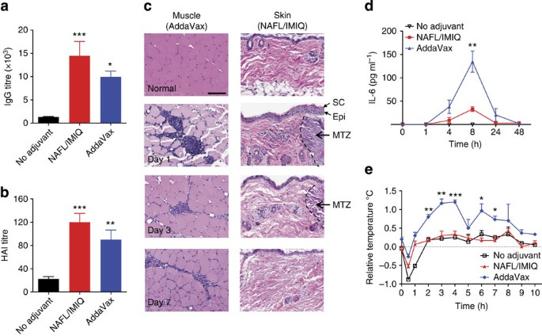Figure 2: Comparison of NAFL/IMIQ with a squalene-based adjuvant. BALB/c mice were ID immunized with influenza vaccine alone (no adjuvant) or in the presence of NAFL/IMIQ adjuvant, or IM immunized with a same dose of the vaccine mixed with squalene-based adjuvant (AddaVax). Serum IgG (a) and HAI (b) levels were measured in 2 weeks.n=8. (c) Haematoxylin and eosin staining of inoculation sites. Muscle and skin tissues of the inoculation sites were collected on days 1, 3 and 7, and shown are representative results of four similar experiments performed. Arrows and black dash lines indicate part of a MTZ. Scale bar, 100 μm. Note: stratum corneum (SC) and epidermis (Epi) are in place after laser treatment. Serum IL-6 was measured at 0, 1, 4, 8, 24 and 48 h after immunization by ELISA (d) and body temperature was monitored hourly for 10 h (e). All temperatures were normalized to non-immunized mice.n=4. Data are presented as mean±s.e.m. Statistical significance was analysed by ANOVA/Bonferroni for (a) and (b), ort-test for (d) and (e). *P<0.05; **P<0.01 or ***P<0.001, respectively. The experiments were repeated twice with similar results, unless noted otherwise. Figure 2: Comparison of NAFL/IMIQ with a squalene-based adjuvant. BALB/c mice were ID immunized with influenza vaccine alone (no adjuvant) or in the presence of NAFL/IMIQ adjuvant, or IM immunized with a same dose of the vaccine mixed with squalene-based adjuvant (AddaVax). Serum IgG ( a ) and HAI ( b ) levels were measured in 2 weeks. n =8. ( c ) Haematoxylin and eosin staining of inoculation sites. Muscle and skin tissues of the inoculation sites were collected on days 1, 3 and 7, and shown are representative results of four similar experiments performed. Arrows and black dash lines indicate part of a MTZ. Scale bar, 100 μm. Note: stratum corneum (SC) and epidermis (Epi) are in place after laser treatment. Serum IL-6 was measured at 0, 1, 4, 8, 24 and 48 h after immunization by ELISA ( d ) and body temperature was monitored hourly for 10 h ( e ). All temperatures were normalized to non-immunized mice. n =4. Data are presented as mean±s.e.m. Statistical significance was analysed by ANOVA/Bonferroni for ( a ) and ( b ), or t -test for ( d ) and ( e ). * P <0.05; ** P <0.01 or *** P <0.001, respectively. The experiments were repeated twice with similar results, unless noted otherwise. Full size image Safety and effectiveness in swine Safety and potency of the adjuvant were further evaluated in swine because porcine skin resembles human skin in term of anatomy, skin reactogenicity, immune responses and pharmacokinetics [20] . Since the skin of pigs is thicker than mice, we used a higher power cosmetic NAFL, named Fraxel SR-1500 (Solta Medical) for pig studies. After one pass of the laser treatment, the pigs were ID vaccinated with 3 μg HA of 2009 H1N1 vaccine, equivalent to a full dose of ID influenza vaccine in humans on the basis of body weight. The immunization enhanced HAI titres by approximately twofold compared with ID vaccine alone ( Fig. 3a ). The laser treatment also increased the production of hepatitis B surface antigen vaccine-specific antibodies by more than five to sevenfold in both primary and booster immunizations ( Supplementary Fig. 6 ). Topical IMIQ further enhanced the immunogenicity in pigs, similarly as described in mice ( Fig. 3a ), but remarkably, concurred with diminished local skin reactogenicity. As shown in Fig. 3b , 1st column, ID influenza vaccine caused wheals with a diameter of 0.5–1 cm right after immunization, concomitant with significant erythema and swelling at the injection site, which peaked on day 3 and resolved by day 7 post immunization, similar to what has been described in humans [21] , [22] . In comparison with influenza vaccine alone, similar or less skin reaction was observed at the injection site immediately (day 0, <30 min) and days 1 and 3 after immunization at laser-treated site ( Fig. 3b 2nd column). Diminished skin irritation was further appreciated on days 1 and 3 by combination of NAFL and IMIQ ( Fig. 3b 4th column), in sharp contrast to the peaking skin irritation seen in the ID group during the same period of time ( Fig. 3b 1st column). The milder skin reactogenicity was measured by 50% reduction in the mean area of erythema at the inoculation site in the NAFL/IMIQ group as compared with the influenza vaccine alone group ( Fig. 3c , 11 versus 23 mm 2 , P <0.001, ANOVA/Bonferroni). In parallel, histology examination of the inoculation sites confirmed drastic diminishment of infiltrated inflammatory cells in pigs receiving influenza vaccine adjuvanted by NAFL/IMIQ as compared with the pigs receiving influenza vaccine alone ( Fig. 3d ). 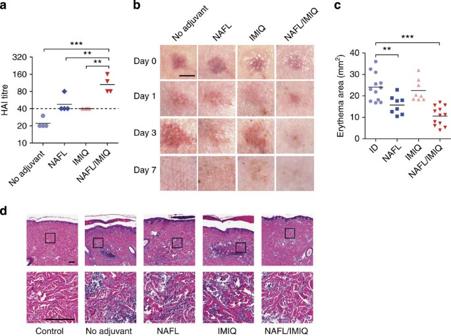Figure 3: NAFL/IMIQ adjuvant in swine study. The exterior hind legs of yorkshire pigs were shaved, cleaned and ID vaccinated with 100 μl of the influenza vaccine (3 μg HA content) only (no adjuvant) or following one pass of laser illumination with Fraxel SR-1500 (NAFL), after which IMIQ was applied to the immunization site (NAFL/IMIQ). Alternatively, the immunization site receiving the vaccine alone was topically applied with IMIQ directly (IMIQ). HAI titres were measured in 2 weeks (a). Each symbol represents data from individual animals, horizontal bars indicate mean, and a dash line marks the standard protective titre of HAI.n=4. (b) Photos were taken right (day 0) and 1, 3 and 7 days after immunization and representative results were shown with four pigs in each group. Scale bar, 5 mm. (c) The erythema areas of injection sites were analysed by Image Pro Premier software 3 days after immunization. Each symbol represents a mean value of one injection site analysed for three times. Horizontal bars indicate the mean. From left to right,n=11, 8, 8 and 12, respectively. (d) Haematoxylin and eosin slides showing infiltrated cells at the inoculation site, representative of six similar results in two separate experiments. Scale bar, 200 μm. Statistical significance was analyzed by ANOVA/Bonferroni. **P<0.01 or ***P<0.001, respectively. Figure 3: NAFL/IMIQ adjuvant in swine study. The exterior hind legs of yorkshire pigs were shaved, cleaned and ID vaccinated with 100 μl of the influenza vaccine (3 μg HA content) only (no adjuvant) or following one pass of laser illumination with Fraxel SR-1500 (NAFL), after which IMIQ was applied to the immunization site (NAFL/IMIQ). Alternatively, the immunization site receiving the vaccine alone was topically applied with IMIQ directly (IMIQ). HAI titres were measured in 2 weeks ( a ). Each symbol represents data from individual animals, horizontal bars indicate mean, and a dash line marks the standard protective titre of HAI. n =4. ( b ) Photos were taken right (day 0) and 1, 3 and 7 days after immunization and representative results were shown with four pigs in each group. Scale bar, 5 mm. ( c ) The erythema areas of injection sites were analysed by Image Pro Premier software 3 days after immunization. Each symbol represents a mean value of one injection site analysed for three times. Horizontal bars indicate the mean. From left to right, n =11, 8, 8 and 12, respectively. ( d ) Haematoxylin and eosin slides showing infiltrated cells at the inoculation site, representative of six similar results in two separate experiments. Scale bar, 200 μm. Statistical significance was analyzed by ANOVA/Bonferroni. ** P <0.01 or *** P <0.001, respectively. Full size image The mechanism of action of NAFL/IMIQ adjuvant To determine the underlying mechanism, we tracked MHC II + cells at the inoculation site with or without laser treatment in mice expressing MHC II infused with green fluorescent protein (GFP) [23] . The MHC II + cells in the skin are mainly DCs, Langerhans cells and macrophages, broadly defined as APCs [24] , [25] . An increase in the motility of APCs was noticed soon after laser treatment and these cells were gradually recruited to the vicinity of MTZs. Their accumulation around individual MTZs became apparent as early as 3 h and peaked 24 h after laser illumination ( Fig. 4a , upper panel). As expected, the MTZ-induced recruitment of APCs was well separated spatially ( Fig. 4a , left panel). To our surprise, IMIQ did not augment, but rather reduced NAFL-induced accumulation of APCs around the MTZs ( Fig. 4a , lower panel), raising a possibility that IMIQ might promote migration of APCs. In an attempt to address this, whole-mount histology of the inoculation site was performed to determine entrances of APCs into lymphatic vessels. It was found that the number of GFP + cells in lymphatic vessels was significantly elevated by IMIQ and to a lesser extent, by NAFL, but it was the combination that led to the highest number of APCs entering into the lymphatic vessels among all the groups at all time points tested ( Fig. 4b,c ). Consistent with the highest number of GFP + cells in the lymphatic vessels was the lowest percentage of CD11c + DCs in the skin, in parallel to a corresponding increase in the number of CD11c + DCs in the draining lymph nodes (dLNs) in mice receiving the vaccine and NAFL/IMIQ adjuvant ( Fig. 4d,e ). Accelerated migration of APCs to dLNs may be crucial on two fronts: (1) augmentation of influenza vaccine-induced immunity and (2) reduction of local inflammation because a smaller number of mature APCs at the inoculation site can facilitate inflammation resolution, whereas a higher number of mature DCs in dLNs are pivotal for heightened immune responses. 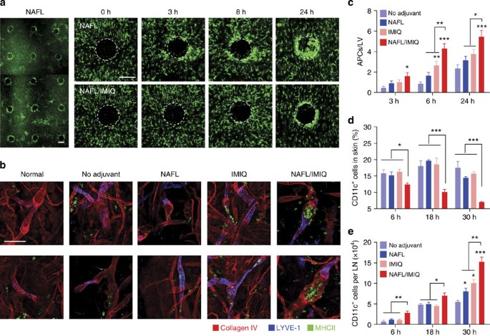Figure 4: Accelerated migration of APCs into dLNs in the presence of NAFL/IMIQ. MHC II-EGFP transgenic mice were ID inoculated in one ear with influenza vaccine adjuvantated with NAFL or NAFL/IMIQ. Accumulation of MHC II+APCs around individual MTZs was visualized by intravital confocal microscopy at varying times after immunization and the one captured at 8 h post immunization was shown ina, left panel. A representative MTZ was tracked at 0, 3, 8 and 24 h after immunization of influenza vaccine with NAFL treatment (upper panel) or NAFL/IMIQ (lower panel) in (a), representative of 6 similar results in two separate experiments. White dash circles highlight MTZs. Scale bar, 200 μm. (b) Monitoring APCs within lymphatic vesseles. Ears were prepared and stained by whole-mount immunohistology 8 h post immunization. APCs (green), lymphatic vessels (blue and/or red) and blood vessels (red) were visualized by confocal microscopy, representative of six similar results in two separate experiments. Scale bar, 100 μm. Average number of APCs within each lymphatic vessel were determined by manual counting GFP+cells inside the lymphatic vessels in 20 randomly selected fields with a total of more than 40 lymphatic vessels counted (c) during which three-D scanning was performed to confirm the intra-vessel localization of each APC (b). (d,e) Proportions of CD11+DCs in the skin (d) and a total number of DCs in each dLN (e). CD11c+DCs in the dorsal skin and dLNs were quantified by flow cytometry at indicated times after immunizing with the influenza vaccine alone or in the presence of indicated adjuvants asFig. 1.n=6, except for NAFL/IMIQ group (n=8). Data are presented as mean±s.e.m. Statistical significance was analysed by ANOVA/Bonferroni. *P<0.05; **P<0.01 or ***P<0.001, respectively. All experiments were repeated twice with similar results. Figure 4: Accelerated migration of APCs into dLNs in the presence of NAFL/IMIQ. MHC II-EGFP transgenic mice were ID inoculated in one ear with influenza vaccine adjuvantated with NAFL or NAFL/IMIQ. Accumulation of MHC II + APCs around individual MTZs was visualized by intravital confocal microscopy at varying times after immunization and the one captured at 8 h post immunization was shown in a , left panel. A representative MTZ was tracked at 0, 3, 8 and 24 h after immunization of influenza vaccine with NAFL treatment (upper panel) or NAFL/IMIQ (lower panel) in ( a ), representative of 6 similar results in two separate experiments. White dash circles highlight MTZs. Scale bar, 200 μm. ( b ) Monitoring APCs within lymphatic vesseles. Ears were prepared and stained by whole-mount immunohistology 8 h post immunization. APCs (green), lymphatic vessels (blue and/or red) and blood vessels (red) were visualized by confocal microscopy, representative of six similar results in two separate experiments. Scale bar, 100 μm. Average number of APCs within each lymphatic vessel were determined by manual counting GFP + cells inside the lymphatic vessels in 20 randomly selected fields with a total of more than 40 lymphatic vessels counted ( c ) during which three-D scanning was performed to confirm the intra-vessel localization of each APC ( b ). ( d , e ) Proportions of CD11 + DCs in the skin ( d ) and a total number of DCs in each dLN ( e ). CD11c + DCs in the dorsal skin and dLNs were quantified by flow cytometry at indicated times after immunizing with the influenza vaccine alone or in the presence of indicated adjuvants as Fig. 1 . n =6, except for NAFL/IMIQ group ( n =8). Data are presented as mean±s.e.m. Statistical significance was analysed by ANOVA/Bonferroni. * P <0.05; ** P <0.01 or *** P <0.001, respectively. All experiments were repeated twice with similar results. Full size image We also found that CD11c + cells only accumulated in ipsilateral, but not in contralateral, lymph nodes indicating that the adjuvant effects of NAFL/IMIQ impacts locally rather than systemically ( Supplementary Fig. 7 ). Therefore, we focused on local events to investigate synergistic adjuvant effects of NAFL and IMIQ. The active recruitment of APCs around each MTZ promoted us to study local chemokine production stimulated by NAFL treatment. Six out of nine chemokines examined were elevated 6 h after NAFL treatment, peaked in 24 h, and dwindled down thereafter ( Fig. 5a ), in agreement with resolving inflammation at the inoculation site in 2 days ( Fig. 2c ). Among these chemokines, CCL2, CCL20, CXCL9, CXCL10, CXCL12 and Chemerin are known to preferably attract pDCs [26] , [27] , [28] , [29] . pDCs, characterized as CD11c + CD11b − B220 + Ly6C + PDCA-1 + cells ( Supplementary Fig. 8a ), accumulated at the inoculation site at a level four times higher after 24 h of NAFL treatment when compared with non-laser-treated skin ( Fig. 5b ). The pDC recruitment was further enhanced by topic IMIQ leading to an eightfold increase in the percentage of pDCs at the inoculation site ( Fig. 5b and Supplementary Fig. 8b ). The pDCs mainly accumulated in the vicinity of MTZs as evidenced by strong immunohistological staining around each MTZ with an antibody against a pDC-specific marker, Siglec H ( Fig. 5c , upper). NAFL/IMIQ might also attract other immune cells, but pDCs were preferable targets of IMIQ because of a high level of TLR-7 expression on the cells [30] . Preferable mobilization of pDCs explained a relatively high level of IFN-α/β, tumour-necrosis factor-α (TNF-α), and IL-6 at the inoculation site 6 h after the immunization in the presence of NAFL/IMIQ adjuvant ( Fig. 5d ), since pDCs, but not conventional DCs, produced high levels of these proinflammatory cytokines on activation by IMIQ ( Supplementary Fig. 9 ). In contrast, IMIQ alone failed to vigorously increase the expression of these cytokines under similar conditions, in agreement with previous investigation [27] . 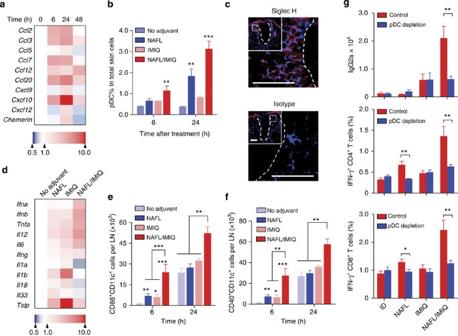Figure 5: NAFL/IMIQ preferably recruits pDCs. (a) Chemokine production at the inoculation site. The levels of indicated chemokines were measured in BALB/c mice after varying times of laser treatment by quantitative real-time PCR (qPCR), normalized to GAPDH and expressed as fold increases relative to time zero. Each square represents the mean value of four mice and colour indicates a fold increase from low (blue) to high (red). (b) Recruitment of pDCs into the inoculation site. pDCs were identified by B220+CD11b−PCDA-1+Ly6C+cells by flow cytometry as described inSupplementary Fig. 6and the percentages of pDCs in total skin cells were determined 6 and 24 h after vaccination with influenza vaccine alone or in the presence of indicated adjuvants.n=4. (c) The inoculation sites were also stained with siglec H-specific antibody (upper panel) or isotype control antibody (lower panel) 24 h after NAFL/IMIQ treatment. Note: Siglec H staining (red) was concentrated around MTZ (white dash lines). Representative results of six similar samples in two separate experiments. Blue, 4',6-diamidino-2-phenylindole staining of cell nuclei. Scale bar, 100 μm. Insets incshow a MTZ (white dash line), part of which is outlined by a white square and enlarged inc. (d) Cytokine expression at the inoculation sites 6 h after immunization. The expression levels of indicated cytokines were measured by qPCR and expressed as fold increases relative to those in the mice receiving no adjuvant. Each square represents a mean of 4 mice. (e,f) Increases in the number of mature DCs in dLNs in mice receiving influenza vaccine and NAFL/IMIQ. dLNs were collected at indicated times after immunization and mature DCs were identified as CD86+CD11c+cells (e) or CD40+CD11c+cells (f).n=6, except for the NAFL/IMIQ group (n=8). (g) Effects of pDC depletion on NAFL/IMIQ-mediated adjuvanticity. Mice were intraperitoneally injected with 400 μg anti-mPDCA-1 antibody or control antibodies (control) at 24 and 0 h before immunization. One week later cellular immune responses were measured (middle and lower panel), and humoral immune responses were measured two weeks later (upper panel).n=8. Data are presented as mean±s.e.m. Statistical significance was analysed by ANOVA/Bonferroni. *P<0.05; **P<0.01 or ***P<0.001, respectively. All experiments were repeated twice with similar results. Figure 5: NAFL/IMIQ preferably recruits pDCs. ( a ) Chemokine production at the inoculation site. The levels of indicated chemokines were measured in BALB/c mice after varying times of laser treatment by quantitative real-time PCR (qPCR), normalized to GAPDH and expressed as fold increases relative to time zero. Each square represents the mean value of four mice and colour indicates a fold increase from low (blue) to high (red). ( b ) Recruitment of pDCs into the inoculation site. pDCs were identified by B220 + CD11b − PCDA-1 + Ly6C + cells by flow cytometry as described in Supplementary Fig. 6 and the percentages of pDCs in total skin cells were determined 6 and 24 h after vaccination with influenza vaccine alone or in the presence of indicated adjuvants. n =4. ( c ) The inoculation sites were also stained with siglec H-specific antibody (upper panel) or isotype control antibody (lower panel) 24 h after NAFL/IMIQ treatment. Note: Siglec H staining (red) was concentrated around MTZ (white dash lines). Representative results of six similar samples in two separate experiments. Blue, 4',6-diamidino-2-phenylindole staining of cell nuclei. Scale bar, 100 μm. Insets in c show a MTZ (white dash line), part of which is outlined by a white square and enlarged in c . ( d ) Cytokine expression at the inoculation sites 6 h after immunization. The expression levels of indicated cytokines were measured by qPCR and expressed as fold increases relative to those in the mice receiving no adjuvant. Each square represents a mean of 4 mice. ( e , f ) Increases in the number of mature DCs in dLNs in mice receiving influenza vaccine and NAFL/IMIQ. dLNs were collected at indicated times after immunization and mature DCs were identified as CD86 + CD11c + cells ( e ) or CD40 + CD11c + cells ( f ). n =6, except for the NAFL/IMIQ group ( n =8). ( g ) Effects of pDC depletion on NAFL/IMIQ-mediated adjuvanticity. Mice were intraperitoneally injected with 400 μg anti-mPDCA-1 antibody or control antibodies (control) at 24 and 0 h before immunization. One week later cellular immune responses were measured (middle and lower panel), and humoral immune responses were measured two weeks later (upper panel). n =8. Data are presented as mean±s.e.m. Statistical significance was analysed by ANOVA/Bonferroni. * P <0.05; ** P <0.01 or *** P <0.001, respectively. All experiments were repeated twice with similar results. Full size image Among these cytokines induced at the inoculation site, TNF-α has been demonstrated to promote migration of dermal DCs into dLNs [31] . We thus ID injected a TNF-α inhibitor, soluble TNF-Receptor Type I (TNF RI) into the inoculation site following the immunization. The TNF-α inhibitor hampered adjuvant effects of NAFL/IMIQ, in particular, on IgG2a production ( P <0.001, t -test), highlighting a critical role for TNF-α in NAFL/IMIQ-mediated adjuvanticity ( Supplementary Fig. 10a ). Moreover, Th1-biased adjuvanticity of NAFL/IMIQ was significantly impaired in mice deficient in interferon regulatory factor 7 (IRF7; Supplementary Fig. 10b , P <0.05 t -test), suggesting contribution of IFN-α/β, two major activators of immature DCs, to the immune enhancement of NAFL/IMIQ as well [32] . This Th1-predominant cytokine milieu at the inoculation site was pivotal for increasing percentages ( Supplementary Figs 11,12a,12b ) and numbers ( Fig. 5e,f ) of CD40 + and CD86 + mature CD11c + DCs in dLNs in the presence of NAFL/IMIQ. The increase in mature DCs was also corroborated with a relatively high mean fluorescent intensity of CD40 and CD86 staining on the cells ( Supplementary Fig. 12a,b ). Notably, the percentages of CD40 + and CD86 + DCs arose significantly in the IMIQ group at 6 or 18 h or in the NAFL group at 6 h after immunization, but the total number of mature DCs in dLNs were much more prominent in the NAFL/IMIQ group, which translated into a strong acquired immunity in the animals ( Fig. 5e,f and Supplementary Fig. 12 ). Strikingly, not all proinflammatory cytokines were synergistically elevated by NAFL/IMIQ, and rather, IL-1 family (IL-1α/β, IL-18, IL-33) and thymic stromal lymphopoietin (TSLP) were diminished considerably as compared with mice immunized with the vaccine alone, or along with either topical IMIQ or NAFL ( Fig. 5d ). The selective decrease in these mediators may be another reason behind a limited local reaction in the presence of NAFL/IMIQ, because both IL-1 family and TSLP are mediators of local inflammation and dermatitis as demonstrated by a number of studies [33] , [34] . To directly address a pivotal role of pDCs in the synergistic adjuvant effect of NAFL and IMIQ, we depleted pDCs in Balb/c mice by injection of anti-mPDCA-1 antibody before immunization [35] . pDC depletion did not affect IgG1 levels, but profoundly impaired IgG2a production in the NAFL/IMIQ group ( Fig. 5g upper panel, P <0.01 t -test). In addition to diminished production of IgG2a, pDC depletion compromised cell-mediated immune responses as well, reflected by significant decreases in the percentages of CD4 + and CD8 + T cells secreting IFN- γ ( Fig. 5g middle and lower panels, P <0.01 t -test). Interestingly, the impairment was not evidenced in the IMIQ group, indicating that the effect of topical IMIQ relied primarily on dermal resident APCs, because pDCs were almost undetectable in normal, non-laser-treated skin [36] . In contrast to IMIQ, pDC depletion resulted in a significant decrease in the percentages of both CD4 + ( P <0.01 t -test) and CD8 + T ( P <0.05 t -test) cells producing IFN-γ in mice immunized with NAFL-adjuvanted influenza vaccine ( Fig. 5g ). The results argue strongly that NAFL-mediated recruitment of pDCs into the inoculation site is key for the observed adjuvant effect of NAFL/IMIQ. Increasing vaccine-induced immune responses in aged mice Given the strong cell-mediated immune response evoked by the new adjuvant, we extended our investigation to old mice, because elderly people respond poorly to current seasonal influenza vaccines. Unfortunately, the elderly suffer from a high level of morbidity and mortality after influenza viral infection and need the vaccine most. As shown in Fig. 6a and Supplementary Fig. 13 , old BALB/c mice elicited a rather weak immune response compared with adult mice after IM immunization with H1N1 influenza vaccine alone. The weak immune response of the old mice was not improved by ID vaccination regardless of whether NAFL or IMIQ was employed. In contrast, the combination of NAFL/IMIQ adjuvant elicited vigorous humoral ( P <0.001, ANOVA/Dunnett’s) and cellular ( P <0.01, ANOVA/Dunnett’s) immune responses in these old animals ( Fig. 6a–c and Supplementary Fig. 13a ). The levels of humoral and cell-mediated responses were arguably greater than those provoked by AddaVax-adjuvanted influenza vaccine or in adult mice IM immunized with the same amount of the influenza vaccine ( Fig. 6a–c , P <0.01, ANOVA/Dunnett’s). Similar to what occurred in adult mice, the NAFL/IMIQ adjuvant increased pDCs in number at the inoculation site and provoked primarily Th1 immune response in old mice as suggested by a higher ratio of IgG2a to IgG1 and greater percentages of IFN-γ-producing CD8 + and CD4 + T cells in the presence versus. the absence of NAFL/IMIQ adjuvant ( Fig. 6b,c , Supplementary Fig. 13b,c ). As a result, ~80% (10/13) of the old mice were protected from lethal H1N1 viral infection after ID immunization of the influenza vaccine with the NAFL/IMIQ adjuvant, which was superior to the 17% (1/6) protection in the mice IM immunized with squalene-adjuvanted influenza vaccine ( Fig. 6d,e ). There was no protection against the viral challenge if the animals were ID immunized with influenza vaccine alone or along with either adjuvant ( Fig. 6d,e ). 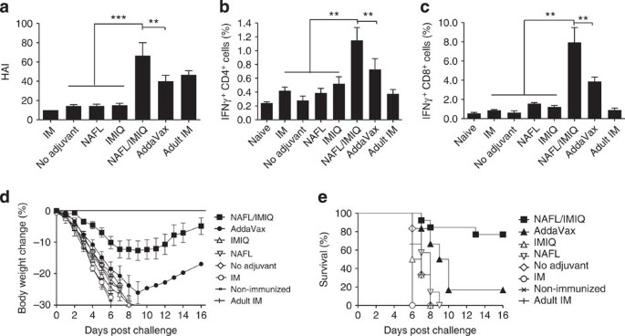Figure 6: NAFL/IMIQ augments protective immunity in old mice. Old BALB/c mice were ID immunized with 0.6 μg (HA content) H1N1 influenza vaccine alone or in the presence of NAFL, IMIQ or NAFL/IMIQ adjuvant. IM immunizations with a same dose of the vaccine mixed with AddaVax adjuvant in old mice or without AddaVax (AddaVax) in both old (IM) and adult (adult IM) mice were used as controls. (a) HAI antibody titres were measured 4 weeks later. Percentages of IFNγ-secreting CD4+(b) and CD8+(c) T cells were analysed in vaccine-stimulated peripheral blood mononuclear cells 1 week after the immunizations. Mice were challenged in 5 weeks with 5 × LD50of mouse-adapted A/California/7/2009 H1N1 viruses. Body weight (d) and survival (e) were monitored daily for 16 days after challenge.n=6, except for the NAFL/IMIQ group (n=13). Data are presented as mean±s.e.m. Statistical significance was analysed by ANOVA/Dunnett’s. **P<0.01 or ***P<0.001, respectively. All experiments were repeated twice with similar results. Figure 6: NAFL/IMIQ augments protective immunity in old mice. Old BALB/c mice were ID immunized with 0.6 μg (HA content) H1N1 influenza vaccine alone or in the presence of NAFL, IMIQ or NAFL/IMIQ adjuvant. IM immunizations with a same dose of the vaccine mixed with AddaVax adjuvant in old mice or without AddaVax (AddaVax) in both old (IM) and adult (adult IM) mice were used as controls. ( a ) HAI antibody titres were measured 4 weeks later. Percentages of IFNγ-secreting CD4 + ( b ) and CD8 + ( c ) T cells were analysed in vaccine-stimulated peripheral blood mononuclear cells 1 week after the immunizations. Mice were challenged in 5 weeks with 5 × LD 50 of mouse-adapted A/California/7/2009 H1N1 viruses. Body weight ( d ) and survival ( e ) were monitored daily for 16 days after challenge. n =6, except for the NAFL/IMIQ group ( n =13). Data are presented as mean±s.e.m. Statistical significance was analysed by ANOVA/Dunnett’s. ** P <0.01 or *** P <0.001, respectively. All experiments were repeated twice with similar results. Full size image Many vaccine adjuvants are being developed in preclinical studies or in various stages of clinical trials and the potency of these conventional adjuvants often comes at the expense of safety [37] . The current investigation explores a novel adjuvant that limits adverse effects locally and systemically, while augmenting efficacy of influenza vaccines in both small and large, young and old animal models. The handheld NAFL device we used is self-applicable and FDA approved for facial wrinkle removal at home, which requires a higher safety standard than laser illumination of a tiny spot on the upper arm used for vaccination in a medical office. The laser parameters in our swine study are well below those normally used in a clinical practice for skin resurfacing, and can be readily incorporated into the existing design of the small device. The 1,410 nm light works in a stamp/scanning fashion and is equally effective regardless of skin colour, in contrast to the 532 nm laser adjuvant described previously [38] , [39] . Its microprobe is tightly sealed by a thin plastic that prevents any skin materials from contaminating the probe, and the sealer is readily cleaned aseptically to prevent person-to-person contamination. The laser does not damage the stratum corneum, the outermost layer of epidermis, so that integrity of the skin barrier is preserved [17] . Another advantage of this adjuvant is its standalone feature, like a topical adjuvant, which means there is no requirement for pre-mixture or reformulation to use it with existing or new vaccines. The adjuvant can also be readily incorporated into portable and/or self-vaccination procedures with various needle-free, painless, microneedle-array patches. IMIQ cream (Aldara) was initially approved by FDA more than 15 years ago as a topical treatment for genital/perianal warts at age 12 or older. The drug has also been approved for the treatment of superficial basal cell carcinoma and actinic keratosis as of 2004. In those treatments, the cream is applied three times a week for up to 12 weeks or daily for several weeks, and in many cases a relatively large area of the skin is affected [19] . In contrast, for use as an adjuvant along with NAFL, IMIQ is topically applied only once to a skin area of smaller than 1 cm 2 , so the systemic absorption or local reaction is extremely limited [40] . In this preclinical study, we showed that a combination of NAFL and topical IMIQ apparently alleviates, rather than worsens, skin irritation provoked by influenza vaccine in pigs. NAFL/IMIQ not only blunts local inflammation but also raises little circulating IL-6 or body fever over influenza vaccines. In contrast, a fever was clearly presented along with a significantly higher level of IL-6 in mice receiving IM vaccination of squalene-adjuvanted vaccines. Whether or not this safer profile demonstrated in mice can translate into humans remains to be investigated. The mechanisms underlying the ability of NAFL/IMIQ adjuvant to augment influenza vaccination while reducing adverse events are likely to be multifaceted. As depicted in Supplementary Fig. 14 , laser-damaged cells in each MTZ release danger signals that stimulate the production of a number of chemokines and preferably attract pDCs from circulation, leading to their increased presence around each MTZ. These pDCs are then activated by IMIQ penetrating from the skin surface because the cells express a high level of TLR-7. On activation, pDCs secrete TNF-α, IFN-α/β and the like, and these cytokines direct maturation and differentiation of APCs in situ , and accelerate trafficking of these mature APCs into dLNs via lymphatic vessels [31] , [32] . Therefore, NAFL-induced recruitment and IMIQ-mediated activation are likely to be the primary mechanisms for the observed synergy of these two adjuvants, resulting in a high level of TNF-α secretion at the inoculation site. An essential part of TNF-α in maturation and migration of dermal DCs into dLNs was clearly demonstrated by the ability of TNF-α inhibitor to impede immune enhancement of NAFL/IMIQ. Moreover, Cumberbatch and Kimber [41] showed that ID injection of TNF-α evoked a concentration and time-dependent maturation and trafficking of dermal DCs into dLNs. On the contrary, mice deficient in TNF-α receptor had impaired DC maturation after bacterial infection [42] . Besides TNF-α, IFN-α/β produced by pDCs also contributed to a high level of Th1 immunity evoked by NAFL/IMIQ. In IRF7 deficient mice whose pDCs could not produce IFN-α/β efficiently [43] , IgG2a production was diminished significantly, in agreement with a recent investigation [44] . Moreover, depletion of pDCs almost completely blunted the adjuvant effect of NAFL/IMIQ on IgG2a production and on cell-mediated immune responses. Another major finding of this investigation is that micro-sterile inflammation induced by NAFL occurs only briefly, peaking at 24 h and subsiding in 48 h, but this short period of local sterile inflammation appears enough to ‘educate’ DCs in bridging an innate to adaptive immune response. These findings are consistent with previous investigations demonstrating that prolonged inflammation induced by alum was dispensable for its adjuvanticity [45] . Surgical removal of the inoculation site containing alum 2 h after vaccination did not affect the adjvuanticity of alum [45] , an argument strongly supported by the current investigation. Besides a shortened period of local inflammation, infiltration of pDCs may also contribute to the reduced skin irritation, as Gregorio et al. [36] reported that pDCs could rapidly infiltrate into skin in response to skin injury, and improve the skin recovery. Finally, a combination of laser and IMIQ selectively reduces the production of the cytokines of the IL-1 family and TSLP that are well known to contribute to the local skin irritation [33] , [34] , which may be another mechanism for reducing local and systemic adverse events of this topical adjuvant. Inflammatory effects of an ideal adjuvant should be localized and transient, which is particularly important for cutaneous vaccination [46] . The finding that a strong immune response can be provoked by transient micro-sterile inflammation at the inoculation site is of highly clinical significance for cutaneous vaccination. A growing body of evidence has shown that cutaneous vaccination is more effective than IM vaccination, as the skin is enriched in APCs and in networks of lymphatic vessels, in contrast to the muscle where few APCs reside. However, severe skin lesions caused by various adjuvants, hamper a broad application of this route of immunization, apart from inconvenience. Therefore, this micro-sterile inflammation-based adjuvant merits clinical investigations for dose-sparing or augmenting the efficacy of influenza vaccines in certain high-risk groups like the elderly. Furthermore, this approach may raise fewer concerns of long-term safety, because only vaccine itself is injected into the body. Animals Inbred BALB/c mice and outbred Swiss Webster mice at 6–8 weeks of age were purchased from Charles River Laboratories. Mice of both genders were used randomly with no notable difference. Eighteen-month-old BALB/c mice (old mice) were purchased from National Institute of Aging (NIA). Irf7−/− mice on C57BL/6J background were a kindly gift of Dr T. Taniguchi, Tokyo University [43] and C57BL/6J control mice were obtained from Jackson Laboratories. MHC II-EGFP mice expressing MHC class II molecule infused into enhanced GFP was a kind gift from Drs Boes and Ploegh, Harvard Medical School [23] . Male Yorkshire pigs at 4 months of age were obtained from the Teaching and Research Resources at Tufts University. The animals were housed in the specific pathogen-free animal facilities of Massachusetts General Hospital (MGH) in compliance with institutional, hospital and NIH guidelines. All studies were reviewed and approved by the MGH Institutional Animal Care and Use Committee. Laser adjuvant A FDA-approved, home-use NAFL laser was used in mice (PaloVia Skin Renewing Laser, Palomar Medical Technologies). The hand held device emits a 1,410-nm laser light and two passes at the medium power were used to generate overlapped MTZs at the inoculation site. Pigs were treated with one pass of Fraxel SR-1500 laser (Solta Medical). This clinical device emitted an array of laser with 17% coverage, 93 MTZs cm −2 per pass and 35 mJ per microbeam. Influenza virus and vaccine Pandemic A/California/7/2009 H1N1 influenza virus was obtained from American Type Culture Collection (ATCC, #FR-201). The virus was expanded in 10-day-old embryonated chicken eggs at 35 °C for 3 days, collected by ultracentrifugation and frozen at −80 °C until use. Its quantity was determined with a 50% tissue culture infectious dose (TCID 50 ) in Madin–Darby canine kidney cells (ATCC, #CCL-34). To challenge mice, the virus was adapted in mice for three cycles of intranasal instillation-lung homogenate preparation and infectivity of the resultant virus was assayed by a 50% lethal dose (LD 50 ) in adult BALB/c mice following a standard protocol. Monovalent A/California/7/2009 H1N1 influenza vaccine (Sanofi Pasteur, Inc.) was obtained from MGH pharmacy and BEI Resources, used at 0.06 μg HA per mouse or 3 μg HA per pig unless otherwise indicated. Immunizations and challenges Mice to be immunized were hair removed on the lower dorsal skin and ID inoculated on the next day with influenza vaccine or illuminated with laser before the vaccine was ID administered. After ID immunization, the inoculation site was either left alone or topically applied with IMIQ (Aldara, 3 M Pharmaceuticals). The inoculation site was then covered with a 3 M Tegaderm film to protect it. For IM injection of adjuvanted influenza vaccine, AddaVax, a squalene-based nano-emulsion adjuvant (Invivogen) with a formulation similar to licensed MF59 adjuvant, was mixed with influenza vaccine at 1:1 ratio and IM injected in a total volume of 20 μl. Body temperature was monitored hourly in some of the mice by a temperature control device (FHC). Blood cytokines were measured by enzyme-linked immunosorbent assay (ELISA) kit (eBiosciences). The immunized and control mice were challenged by intranasal instillation of 10 × LD 50 mouse-adapted 2009 H1N1 viruses. Body weight and survival were monitored daily for 14 days unless otherwise specified. In some infection experiments, lungs were collected 4 days after challenge to measure lung viral titres by TCID 50 assays. To immunize pigs, the animals were anaesthetised by IM injection of telazol (2.2 mg kg −1 )/xylazine (2.2 mg kg −1 )/atropine (0.04 mg kg −1 ) and maintained under isoflurane (2–3%) inhalation during hair removal and immunization. Immunization procedure was similar as described in mice with 100 μl influenza vaccine (3 μg HA content) inoculated into the exterior hind leg skin either alone or in the presence of NAFL, IMIQ, or NAFL/IMIQ adjuvant. To quantify local skin reactions, the inoculation sites were photographed and the erythema area at each inoculation site was circled and analysed by Image Pro Premier software (Media Cybernetics, Inc) for three times with which mean erythema area of each inoculation site was calculated. HAI assay HAI titres were assayed according to a published protocol (PMID: 19274084). Serum samples were incubated with receptor-destroying enzyme (Denka Seiken) at 37 °C overnight followed by heat inactivation at 56 °C for 30 min. The resultant serum samples were incubated with four HA units of influenza virus at 37 °C for 1 h after serial dilutions, and then with 0.5% chicken red blood cells (Charles River Laboratories) at room temperature for 30 min. The HAI titre was defined as the reciprocal of the highest dilution that inhibited HA. ELISA Vaccine-specific IgG, IgG1, IgG2a and IgA antibody titres were measured by ELISA. In brief, 1 μg ml −1 recombinant HA was coated onto ELISA plates in NaHCO 3 buffer, pH9.6. After incubation with serially diluted serum samples, HRP-conjugated goat anti-mouse IgG (NA931V, GE Healthcare, dilution 1:6,000), IgG1 (A90-105P, Bethyl, dilution 1:10,000), IgG2a (61-0220, Life Technologies, dilution 1:2,000) or IgA (A90-103P, Bethyl, 1:10,000) antibody was added to measure specific subtypes. For C57BL/6 mice, anti-mouse IgG2c (1079-05, Southern Biotech, 1:5,000) antibody was used in place of anti-IgG2a antibody. Cell-mediated immune responses One week after immunization, blood samples were collected from immunized and control mice in a heparinized tube by tail vein bleeding. Peripheral blood mononuclear cells were isolated after red blood cell lysis. Peripheral blood mononuclear cells (10 6 cells per ml) were incubated with influenza vaccine (1 μg ml −1 HA content) and anti-CD28 (clone 37.51, BD Pharmingen, 4 μg ml −1 ) antibody overnight. Golgi-Plug (BD Pharmingen) was added to prevent cytokine secretion in the final 5 h of the incubation. The stimulated cells were stained with fluorescence-conjugated antibodies against CD4 (clone RM4-5, Biolegend, dilution 1:100), CD8 (clone 53-6.7, Biolegend, dilution 1:200) and IFNγ (clone XMG1.2, Biolegend, 1:100), followed by flow cytometric analysis as previously reported [47] . Histological examination Mice were ID immunized with influenza vaccine in the presence of NAFL/IMIQ adjuvant or IM with the vaccine mixed with AddaVax. The tissues at the inoculation site were dissected at indicated days, fixed and stained by a standard haematoxylin and eosin procedure. Similar histological examination was also carried out in pigs after 3 days of immunization. The slides were scanned and analysed by NanoZoomer (Hamamatsu). Intravital confocal imaging The ear of MHC II-EGFP transgenic mice was treated by NAFL or NAFL/IMIQ. GFP + cells in the epidermis and dermis were imaged by intravital two-photon confocal microscopy (Olympus FV-1000). Three-D reconstruction was used to visualize accumulation of GFP + cells around individual MTZs by Image J software. Whole-mount immune histology The ear of MHC II-EGFP transgenic mice was inoculated with influenza vaccine in the presence of the indicated adjuvants. The outer ear flaps were prepared at indicated times post immunization, fixed by 4% formaldehyde at 4 °C overnight and blocked by 2% fetal bovine serum/PBS for 2 h at room temperature. The fixed samples were reacted with rat anti-LYVE-1 (clone 223322, R&D systems, 8 μg ml −1 ) antibody to identify lymphatic vessels and rabbit anti-Collagen IV (ab6586, Abcam, 10 μg ml −1 ) antibody at 4 °C overnight to label both lymphatic and blood vessels, after which the samples were stained with Cy3-conjugated anti-rat (A10522, Life Technology, dilution 1:100) and NL637-conjugated anti-rabbit (NL005, R&D systems, dilution 1:100) antibodies at 4 °C overnight. The stained samples were mounted and imaged by two-photon confocal microscopy (Olympus FV-1000). Immunohistological analysis of pDCs The lower dorsal skin of mice was exposed to NAFL/IMIQ adjuvant. Twenty-four hours later, full thickness of the skin at the site of laser illumination was excised, and frozen tissue sections were prepared and labelled by anti-mouse Siglec H (clone 440c, eBioscience, 10 μg ml −1 ) or isotype control antibody followed by staining with DL594-conjugated goat anti-rat IgG (SA5-10081, Thermo Pierce, dilution 1:100) antibody. The slides were mounted with a mount medium containing a nuclear staining fluorescence dye of 4',6-diamidino-2-phenylindole and imaged by confocal microscopy. Analysis of dermal DCs or pDCs by flow cytometry Skin at the inoculation site was excised, minced and digested with Dispase II (Life Technologies) and Collagenase D (Roche) for 2 h at 37 °C. The digested skin tissues were passed through a 100-μm cell strainer to prepare single-cell suspensions. The resultant cells were treated with anti-CD16/CD32 antibody (clone 93, Biolegend, dilution 1:50) for 20 min, followed by staining with the following fluorescence-conjugated antibodies for 30 min on ice: APC-anti–PDCA-1(clone 927, dilution 1:300), PE-anti- CD11c (clone N418, eBiocience, dilution 1:100), BV421-anti-CD11b (clone M1/70, dilution 1:100), FITC-anti-MHCII (clone M5/114.15.2, dilution 1:200), FITC- anti-Ly6C (clone HK1.4, dilution 1:200), and APC/Cy7-anti-B220 (clone RA3-6B2, dilution 1:100). All antibodies were purchased from Biolegend unless otherwise stated. The stained cells were acquired on a FACSAria (BD) and analysed using FlowJo software (Tree Star). In vivo depletion of pDCs Balb/c mice were intraperitoneally injected with two doses of anti-mPDCA-1 antibody (clone JF05-1C2.4.1, Miltenyi Biotec) at 400 μg per dose at 24 and 0 h, respectively, before immunization [35] . Depletion efficiency was confirmed by flow cytometry of pDCs in the blood samples. Effects of pDC depletion on cellular immune responses were evaluated one week later, and humoral immune responses were analysed 2 weeks after the immunization. Quantification of DCs in dLNs dLNs were collected and single-cell suspensions were prepared, counted, stained with FITC-anti-CD11c (clone N418, eBiociences, dilution 1:100), APC-anti-CD40 (clone 3/23, Biolegend, dilution 1:100) and PerCp-Cy5.5-anti-CD86 (clone GL-1, Biolegend, dilution 1:100) antibodies, followed by flow cytometry. Total numbers of CD11c + cells, CD40 + CD11c + cells or CD86 + CD11c + cells per lymph node were calculated in the basis of the total number of cells and percentages of each cell subset in the lymph node. Quantitative real-time PCR To analyse chemokine and inflammatory cytokine expression at the inoculation site, the full thickness of the skin area about 7 × 10 mm 2 was excised, and total RNA was extracted, reverse-transcribed and amplified by qPCR using a SYBR Green PCR kit (Roche). GAPDH was used as an internal control. All genes and their primers were listed in Supplementary Table 1 . Statistical analysis Two-tailed t -test ( t -test) was used to analyse a difference between two groups, and one-way ANOVA was used among multiple groups. ANOVA followed by Bonferroni correction (ANOVA/Bonferroni) was used to compare selected pairs, and ANOVA followed by Dunnett’s test (ANOVA/Dunnett’s) was for comparing all groups with a control group. P -value was calculated by PRISM software (GraphPad) and a difference was regarded significant if P -value was less than 0.05. Sample sizes were designed based on preliminary experiments to give statistical power. No animals were excluded from the analysis. The investigators were not blinded to the experiments, which were carried out under highly standardized and predefined conditions, except for photo analysis and haematoxylin and eosin slide examination that were performed in an investigator-blind fashion. How to cite this article: Wang, J. et al. A micro-sterile inflammation array as an adjuvant for influenza vaccines. Nat. Commun. 5:4447 doi: 10.1038/ncomms5447 (2014).